Active control of magnetoresistance of organic spin valves using ferroelectricity Organic spintronic devices have been appealing because of the long spin lifetime of the charge carriers in the organic materials and their low cost, flexibility and chemical diversity. In previous studies, the control of resistance of organic spin valves is generally achieved by the alignment of the magnetization directions of the two ferromagnetic electrodes, generating magnetoresistance. Here we employ a new knob to tune the resistance of organic spin valves by adding a thin ferroelectric interfacial layer between the ferromagnetic electrode and the organic spacer: the magnetoresistance of the spin valve depends strongly on the history of the bias voltage, which is correlated with the polarization of the ferroelectric layer; the magnetoresistance even changes sign when the electric polarization of the ferroelectric layer is reversed. These findings enable active control of resistance using both electric and magnetic fields, opening up possibility for multi-state organic spin valves. Since the pioneering work by Dediu et al. [1] and Xiong et al. [2] , many of the follow-up studies have focused on achieving high magnetoresistance (MR) in organic spin valves (OSVs) and uncovering the underlying transport mechanisms [3] , [4] , [5] , [6] , [7] , [8] , [9] , [10] , [11] . It has been generally acknowledged that the interfaces between the organic layer and the ferromagnetic electrodes play a critical role in determining the actual spin-dependent transport mechanism [12] , [13] , [14] , [15] . Barraud et al. [16] studied the spin transport of an OSV in which the thin organic layer serves as a tunnelling barrier as opposed to a diffusive spacer. A spin transport model describing the role of interfacial spin-dependent metal/organic hybridization on the amplitude and sign of the MR was put forward [16] , [17] . Recently, Schulz et al. [18] observed a reversal of the spin polarization of extracted charge carriers by introducing a thin interfacial permanent dipolar layer (LiF). This work indicates that the local electric dipole moment at the interface is important for MR, although in such a device the added dipolar layer plays only a passive role in terms of controlling MR. In the following, we employ a ferroelectric (FE) thin interfacial layer between the organic semiconductor and the ferromagnetic electrode in OSV to achieve active control of MR. The material of choice for the FE layer is PbZr 0.2 Ti 0.8 O 3 (PZT), which has a large polarization (~80 μC cm −2 ) [19] . The PZT layer can induce strong interfacial dipoles and built-in electric field between the organic spacer layer and the ferromagnetic electrode. The interfacial dipole is switchable by external electric field, potentially allowing the control of the spin polarization of injected carriers in organic spintronics. We show that the resistance can be controlled by not only the spin alignment of the two ferromagnetic electrodes [3] , but also by the electric polarization of the PZT layer. The sign of MR changes when electric polarization of the PZT layer is reversed. This new tunability can be understood in terms of the change of relative energy level alignment between ferromagnetic electrode and the organic spacer caused by the electric dipole moment of the FE layer. Device structure and characterizations of the PZT films Our fabricated OSVs consist a 65-nm Alq 3 (tris-(8-hydroxyquinoline) aluminum) layer sandwiched between a 5-nm-thick PZT layer epitaxially grown on a 30-nm-thick La 0.67 Sr 0.33 MnO 3 (LSMO) film-buffered SrTiO 3 (STO) substrate, and a 10-nm-thick (nominal thickness) cobalt layer with gold capping. In this LSMO/PZT/Alq 3 /Co junction (FE-OSV), Co and LSMO serve as the top and bottom magnetic electrodes, respectively. The device structure is schematically shown in Fig. 1a . As discussed in the following, such kind of devices exhibit striking tunability, that is, both the amplitude and sign of MR are tunable due to the presence of the FE PZT. 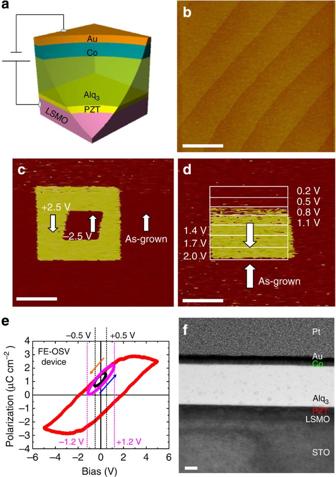Figure 1: Structure of the organic spin valves and characterization of ferroelectricity in the epitaxial PZT. (a) Schematic structure of a Au/Co/Alq3/PZT/LSMO organic spin valve (FE-OSV). (b) Atomic force microscopy topography image of a PZT layer (5 nm in thickness) epitaxially grown on a LSMO (30 nm)/STO substrate. (c) PFM (phase) response measured after successively switching the polarization of the PZT film by applying +2.5 V and −2.5 V on the tip with respective to the LSMO bottom electrode. Note that the protocol of voltage polarity is different in PFM measurements from that in resistance measurements. (d) PFM image showing the polarization reversal by gradually increasing the applied voltage. The ‘up’ (‘down’) arrow corresponds to the polarization pointing out of (into) the film surface. Scale bar, 500 nm (b–d). (e) A typical polarization-voltage loop for the FE-OSV (device A). The black and pink circles illustrate the ‘minor loops’ corresponding toVMAXof ±0.5 and ±1.2 V, respectively. The orange (blue) arrow indicates the direction of the ramp voltage: sweeping down (up) before the MR scans. (f) TEM image for FE-OSV device. Different layers can be distinguished as labelled. Scale bar, 20 nm. Figure 1: Structure of the organic spin valves and characterization of ferroelectricity in the epitaxial PZT. ( a ) Schematic structure of a Au/Co/Alq 3 /PZT/LSMO organic spin valve (FE-OSV). ( b ) Atomic force microscopy topography image of a PZT layer (5 nm in thickness) epitaxially grown on a LSMO (30 nm)/STO substrate. ( c ) PFM (phase) response measured after successively switching the polarization of the PZT film by applying +2.5 V and −2.5 V on the tip with respective to the LSMO bottom electrode. Note that the protocol of voltage polarity is different in PFM measurements from that in resistance measurements. ( d ) PFM image showing the polarization reversal by gradually increasing the applied voltage. The ‘up’ (‘down’) arrow corresponds to the polarization pointing out of (into) the film surface. Scale bar, 500 nm ( b – d ). ( e ) A typical polarization-voltage loop for the FE-OSV (device A). The black and pink circles illustrate the ‘minor loops’ corresponding to V MAX of ±0.5 and ±1.2 V, respectively. The orange (blue) arrow indicates the direction of the ramp voltage: sweeping down (up) before the MR scans. ( f ) TEM image for FE-OSV device. Different layers can be distinguished as labelled. Scale bar, 20 nm. Full size image After epitaxial growth of PZT on LSMO/STO, the PZT layer has a smooth surface with atomically flat terraces, as characterized by atomic force microscopy shown in Fig. 1b . This provides an ideal base for preparing a well-defined Alq 3 /PZT interface. The purpose of introducing the 5-nm-thick-PZT is to tune the energy level alignment between the Alq 3 and LSMO layers because the polarization in PZT is switchable by applying an electric field. Therefore, the polarization reversal of the PZT is crucial. Here we have characterized the polarization reversal of the PZT films used in the FE-OSV devices with piezoelectric force microscopy (PFM). Figure 1c shows a PFM image of the PZT film with a part of the film poled by a conducting tip with ±2.5 V relative to the LSMO bottom electrode. It shows that the polarization of the as-grown films is pointing ‘up’, and a clear reversal of polarization between ‘up’ and ‘down’ states can be created by sign reversal of the applied voltage. Figure 1d shows the voltage dependence of the polarization. It is clear that the polarization of the PZT film (5 nm in thickness) starts to switch to the ‘down’ state when the voltage of the scanning probe exceeds 0.8 V. The polarization reversal of the PZT in the FE-OSV is characterized by the measurements of the hysteretic polarization-voltage dependence. As shown in Fig. 1e , with the Alq 3 /Co/Au layers on top of PZT, the coercive voltage is ~2 V. Figure 1f shows the transmission electron microscope (TEM) image for the cross-section of the FE-OSV. No significant diffusion of Co atoms into the Alq 3 layer is observed (see Supplementary Fig. 1 and Supplementary Note 1 ). Hysteretic behaviour of the MR It has been known that MR depends sensitively on the measuring voltage ( V MR ). Previous studies indicated that MR of LSMO/Alq 3 /Co junctions (LSMO-OSV) increases with decreasing V MR , reaching a maximum when V MR is close to zero [2] , [16] . For our FE-OSV junctions, its MR depends not only on V MR , but also on the history of the voltage applied, giving rise to a strong hysteretic behaviour. We characterize this hysteretic behaviour by measuring MR ( V MR ) profile after applying a ramping voltage ( V MAX ) that is larger than V MR (see Supplementary Fig. 2 and Supplementary Note 2 for the detailed measurement protocol). As shown in Fig. 2 , for a FE-OSV containing an as-grown PZT layer, the MR (at T =11 K) is always negative and is the largest when V MR is near zero, which is similar to numerous previous studies on LSMO-OSV [2] , [4] , [5] , [6] , [8] , [9] , [10] , [11] . The different features in the FE-OSV are: (1) the MR( V MR ) profile is strongly affected by the initial voltage ( V MAX ) and (2) a positive (negative) V MAX leads to a negative (positive) shift of the MR( V MR ) profile along the V MR axis ( Fig. 2d,e ). This shift (Δ V ) is closely tied to the hysteretic behaviour of the PZT layer (so-called minor loops, see Fig. 1e ) and increases with increasing V MAX , as shown in Fig. 2f . The switching fields, MR uncertainty and MR loops reproducibility in FE-OSVs are shown in Supplementary Figs 3–5 and Supplementary Notes 3 and 4 , respectively. 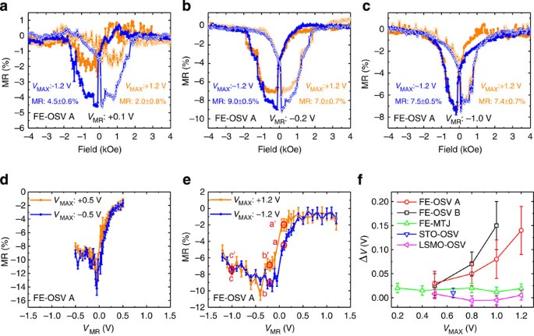Figure 2: Hysteretic behaviour of the MR atT=11 K. (a–c) MR scans in the as-grown state of a FE-OSV device (PZT in ‘up’ polarization) with the same applied bias (VMR) but different initial ramping voltage (VMAX). Here, LSMO is treated as the anode. The switching fields of FE-OSV are confirmed by superconducting quantum interference device measurements (seeSupplementary Fig. 3andSupplementary Note 3). (d,e) MR(VMR) profiles taken at two different values of positive (orange) and negative (blue)VMAX. ΔVrepresents the shift of MR (VMR) profiles, anda′/a,b′/bandc′/cmark the positions at which the six MR loops ina–care taken(VMAX: +1.2 V and −1.2 V). (f) Dependence of ΔVonVMAX. ΔVfor both FE-OSV devices (A and B) increases with increasingVMAX, while the three types of control devices (FE-MTJ, STO-OSV and LSMO-OSV) do not show any significant ΔV. The error bars represent the uncertainty of the MR measurements including both systematic error (estimated from the asymmetry in the MR loops) and the statistical error (seeSupplementary Fig. 4andSupplementary Note 4). Figure 2: Hysteretic behaviour of the MR at T =11 K. ( a – c ) MR scans in the as-grown state of a FE-OSV device (PZT in ‘up’ polarization) with the same applied bias ( V MR ) but different initial ramping voltage ( V MAX ). Here, LSMO is treated as the anode. The switching fields of FE-OSV are confirmed by superconducting quantum interference device measurements (see Supplementary Fig. 3 and Supplementary Note 3 ). ( d , e ) MR( V MR ) profiles taken at two different values of positive (orange) and negative (blue) V MAX . Δ V represents the shift of MR ( V MR ) profiles, and a ′ /a , b ′ /b and c ′ /c mark the positions at which the six MR loops in a – c are taken( V MAX : +1.2 V and −1.2 V). ( f ) Dependence of Δ V on V MAX . Δ V for both FE-OSV devices (A and B) increases with increasing V MAX , while the three types of control devices (FE-MTJ, STO-OSV and LSMO-OSV) do not show any significant Δ V . The error bars represent the uncertainty of the MR measurements including both systematic error (estimated from the asymmetry in the MR loops) and the statistical error (see Supplementary Fig. 4 and Supplementary Note 4 ). Full size image The hysteretic behaviour of the MR was not observed in OSVs without the FE layer, including a conventional LSMO/Alq 3 /Co OSV (LSMO-OSV) and a LSMO/STO/Alq 3 /Co OSV (STO-OSV) in which the 5-nm PZT is replaced by 5-nm STO (see Supplementary Figs 6 and 7 , and Supplementary Note 5 for detailed MR loops and MR ( V MR ) profiles). This indicates that the hysteretic behaviour of the MR in FE-OSV is tied to the presence of PZT. The distinctly different behaviour between the FE-OSV and the PZT-free OSVs (LSMO-OSV and STO-OSV) also allow us to exclude the possibility of resistive bistability mechanism caused by the existence of the trap states or current conduct path inside the Alq 3 layer [20] , [21] , as otherwise similar MR behaviour should be observed in both types of devices. We have also performed measurements on a LSMO/PZT/Co magnetic tunnel junction (FE-MTJ, see Supplementary Fig. 8 ). Although V MAX affects the MR ( V MR ) profile, which confirms the results of Pantel et al. [22] and Valencia et al. [23] , it does not induce any shift of the MR ( V MR ) profile along the V MR axis. The comparison of the MR ( V MR ) profiles of the FE-OSV and the FE-MTJ suggests that the effective voltage generated by the dipole of the PZT (instead of the interfacial bonding) is responsible for the hysteretic behaviour of the MR in the FE-OSV. The FE-MTJ does not show hysteretic behaviour of MR, because no direct dipole exists on the surface of the PZT due to the screening effect from the two metal electrodes in direct contact with the PZT layer. A schematic model is illustrated in Fig. 3 to explain this hysteretic behaviour of MR in the FE-OSV. When a V MAX is applied to the junction, the polarization of the PZT gets modified. Owing to the dipole moment created by the electric polarization of PZT, the effective voltage V eff applied on the Alq 3 layer equals V MR + Δ , where Δ is the vacuum level shift caused by the remnant dipole moment of PZT. When a positive (negative) V MAX is applied, Δ becomes larger (smaller), which explains why the MR ( V MR ) profile can be shifted by V MAX . 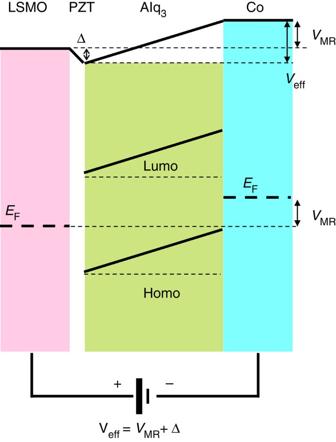Figure 3: Model of the hysteretic behaviour in FE-OSV. The relation between the effective bias on the spacer Alq3(Veff), the applied bias at measurement (VMR) and the vacuum level shift (Δ) by the remanent dipole moments of the FE PZT layer, isVeff=VMR+Δ. Figure 3: Model of the hysteretic behaviour in FE-OSV. The relation between the effective bias on the spacer Alq 3 ( V eff ), the applied bias at measurement ( V MR ) and the vacuum level shift (Δ) by the remanent dipole moments of the FE PZT layer, is V eff = V MR +Δ. Full size image Switch of the MR sign Remarkably, a reversal of the polarization of the PZT layer leads to a sign change of the MR in the FE-OSV. After measuring the MR and MR ( V MR ) profile ( Fig. 4a–c ) for the FE-OSV device B (PZT layer in the as-grown state), we measured polarization-voltage dependence up to ±5 V. The measurement ended at −5.0 V to pole the PZT to the ‘down’ state. The MR measurements of the FE-OSV device after this treatment are shown in Fig. 4d,e,g,h . The shape of the MR ( V MR ) profile changes dramatically, as shown in Fig. 4i . In particular, the sign of the MR changes from negative ( Fig. 4a,b ) to positive ( Fig. 4d,g,h ) for a certain range of V MR . A close correlation between the polarization of PZT and the sign of the MR can be identified by comparing the hysteretic behaviour of the MR ( V MR ) profile and the possible minor polarization-voltage loop of the PZT, as illustrated in Fig. 4f , that is, when the polarization of PZT is negative enough (more ‘down’ state), the MR becomes positive. 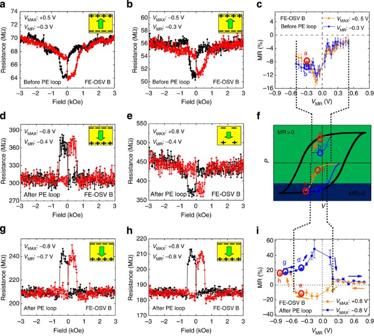Figure 4: Reversal of MR sign atT=11 K. (a,b) MR scans for the ‘as-grown’ state of the FE-OSV device B acquired atVMR=−0.3 V/VMAX=+0.5 V andVMR=−0.3 V/VMAX=−0.5 V, respectively. (c) MR (VMR) profiles atVMAX=+0.5 V (orange) and −0.5 V (blue). (d,e,g,h) MR scans taken when the polarization of the PZT is reversed. (f) Comparison of the MR (VMR) profile and the polarization-voltage loop, illustrating the correlation between the sign of MR and the polarization of the PZT. The asymmetric regions of MR<0 and MR>0 in polarization-voltage loop indicate that the reversal of MR only occurs at higher degree of polarization in the ‘down’ state of PZT. (i) MR(VMR) profiles atVMAX: ±0.8 V when the polarization of the PZT is reversed. The red (blue) circles indicate theVMRvalues at which the MR loops (a,b,d,e,g,h) are taken with positive (negative)VMAX. The error bars are estimates using the same analysis as that inFig. 2. Figure 4: Reversal of MR sign at T =11 K. ( a , b ) MR scans for the ‘as-grown’ state of the FE-OSV device B acquired at V MR =−0.3 V/ V MAX =+0.5 V and V MR =−0.3 V/ V MAX =−0.5 V, respectively. ( c ) MR ( V MR ) profiles at V MAX =+0.5 V (orange) and −0.5 V (blue). ( d , e , g , h ) MR scans taken when the polarization of the PZT is reversed. ( f ) Comparison of the MR ( V MR ) profile and the polarization-voltage loop, illustrating the correlation between the sign of MR and the polarization of the PZT. The asymmetric regions of MR<0 and MR>0 in polarization-voltage loop indicate that the reversal of MR only occurs at higher degree of polarization in the ‘down’ state of PZT. ( i ) MR( V MR ) profiles at V MAX : ±0.8 V when the polarization of the PZT is reversed. The red (blue) circles indicate the V MR values at which the MR loops ( a , b , d , e , g , h ) are taken with positive (negative) V MAX . The error bars are estimates using the same analysis as that in Fig. 2 . Full size image The physical origin of MR sign of the LSMO/Alq 3 /Co junctions has been studied previously by Barraud et al. [16] using nanoindentation-based devices. It was argued that first, the spin polarization alignment P * at the Co/Alq 3 interface [16] is positive when electrons move from Co to Alq 3 , that is, P *(Alq 3 →Co)>0 where the arrow indicates the direction of the electric current [4] , [24] ; second, the density of states for Alq 3 at the Alq 3 /LSMO interface is spin polarized due to the coupling between the two materials, causing P *(LSMO→Alq 3 )<0 when the Alq 3 serves as a diffusive spacer [16] . Following these arguments, Barraud et al. [16] concluded that the sign of MR at small measurement voltages is determined by the sign of the product of P *(Alq 3 →Co) and P *(LSMO→Alq 3 ); the result is negative. In the FE-OSV studied here, the P *(Alq 3 →Co)>0 can be assumed similarly; the polarization alignment P * between LSMO and Alq 3 is not changed by inserting a thin layer (5 nm) of as-grown PZT or STO, but can be changed by poling the PZT layer, according to the behaviour of the observed MR. This novel feature in FE-OSV must be due to the more complex LSMO/PZT→Alq 3 interface. We propose the following model based on the relative energy level alignment between Alq 3 and LSMO to understand the switching of MR sign in FE-OSV. Here we consider mainly the hole transport, because for Alq 3 the energy difference between the highest occupied molecular orbital (HOMO) and Fermi levels of the two metallic LSMO and Co electrodes are much smaller than that between the lowest unoccupied molecular orbital and the Fermi levels [2] , [18] , [25] . As shown in Fig. 5a , when the polarization of the PZT layer is pointing ‘up’ (the as-grown state) or zero (the same case as for STO), the hole injection from the LSMO electrode for positive V MR is from the Fermi level (which lies in the spin majority band) of LSMO to the HOMO of Alq 3 , which is the same as in the LSMO-OSV. Therefore, P *(LSMO/PZT→Alq 3 )<0, corresponding to a negative MR considering P *(Alq 3 →Co)>0 as discussed above [2] , [4] . When the polarization of the PZT layer is pointing ‘down’, the HOMO of A1q 3 is shifted up due to the dipole moment of PZT. Therefore, another state of the LSMO with opposite spin polarization may be accessible ( Fig. 5b ). Hence, P *(LSMO/PZT→Alq 3 ) changes the sign and becomes positive, corresponding to a reversed, positive MR. 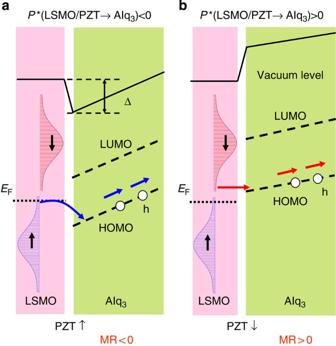Figure 5: Model of MR sign reversal in FE-OSV. (a,b) The energy diagrams of the FE-OSV device when the electric polarization of the PZT is ‘up’ and ‘down’, respectively. The white circles represent the injected holes in the device. The blue (red) arrows indicate the injection of spin-polarized holes from the majority (minority) band of LSMO. Figure 5: Model of MR sign reversal in FE-OSV. ( a , b ) The energy diagrams of the FE-OSV device when the electric polarization of the PZT is ‘up’ and ‘down’, respectively. The white circles represent the injected holes in the device. The blue (red) arrows indicate the injection of spin-polarized holes from the majority (minority) band of LSMO. Full size image Our proposed model relies on two key assumptions: (1) the dipole moment of the PZT layer shifts the Alq 3 HOMO level and (2) the shift of the Alq 3 HOMO level results in a shift of the initial state of LSMO for the hole injection between energy band of opposite spin polarizations. The first assumption was used by Schultz et al. [18] to explain the MR sign reversal in a FeCo/Alq 3 /LiF/NiFe junction by proposing a shift of the HOMO of Alq 3 due to the dipole moment of LiF layer. The second assumption can be justified by the half metallicity of LSMO. As illustrated in Fig. 5 , the conduction band of LSMO splits into spin majority and minority bands due to the exchange interaction, causing half metallicity because the Fermi level lies within the fully polarized spin majority band [26] , [27] , [28] . Therefore, when the HOMO of Alq 3 is shifted up due to the reversal of dipole moment of PZT, the initial state of LSMO for hole injection may change to spin minority band with opposite spin polarization. Note that this reversed dipole moment of PZT needs to be large enough to shift the HOMO level of Alq 3 to ‘reach’ the spin minority band of LSMO and obtain reversed positive MR values. Otherwise, only negative MR values will be observed, as shown in Fig. 4f (also see Supplementary Fig. 9 and Supplementary Note 6 ). Besides changing the energy level alignments, switching the electric polarization of the FE layer may also modify the coupling between the FE layer and the magnetic electrode, depending on the detailed electronic structure of the electrode and the nature of the electric polarization of the FE material [29] , [30] , [31] . These effects may also change the spin polarization at the interface between the FE material and the metal electrode [22] , [23] , [31] . However, both the magnetic structure of the LSMO and the spin polarization of the PZT are not expected to be affected very much by the electric polarization of the PZT, because of the robust magnetic properties of the La 0.7 Sr 0.3 MnO 3 with given composition (far from the metal-insulator phase boundary) and the large distance between the Mn site from LSMO and Ti sites from PZT at the interface [22] , [23] , [30] , [31] . Another possible scenario involves the change of carrier type when the energy level alignment between LSMO and Alq 3 is changed: the carriers take the path of the HOMO (lowest occupied molecular orbital),that is, hole (electron) transport in Alq 3 when the energy levels of Alq 3 is shifted ‘down’ (‘up’) due to the ‘up’ (‘down’) polarization of the PZT layer. This, however, contradicts our experimental observations because in the FE-OSV with the as-grown (‘up’ polarization) PZT, the MR is negative, the same as that in the STO-OSV or LSMO-OSV without any interfacial layers, suggesting that the carrier type in FE-OSV is most probably holes instead of electrons [18] , [25] , as in the STO-OSV or LSMO-OSV. The active control of the energy level alignment between the electrodes and the organic material, manifested here in the active control of the MR, not only carries promises for multistate control of organic spin-valve devices, but will also impact other organic electronic devices, in particular those applied in photovoltaics and solid-state lighting. Specifically, the charge carrier injection efficiency of the organic light emitting diode is determined by the relative alignment between the Fermi energy of the electrode and the energy levels of the organic material [32] . The charge collection efficiency in an organic photovoltaic device also depends on the alignment of the energy levels of the acceptor organic material and the electrode [33] . Therefore, the realization of the active control of the level alignment using an FE interfacial layer demonstrated in this letter may also lead to successful optimization of other organic electronic devices by tailoring the energy landscape of the comprising materials using a tunable interfacial layer. Device fabrication PZT (5 nm), STO (5 nm) and LSMO (30 nm) thin films epitaxially grown on STO (001) substrate by pulsed laser deposition were fabricated into bottom electrodes using conventional wet-etching photolithography [11] , [34] . The Alq 3 (99.995%, Aldrich) layer (thickness: 65 nm) was deposited by thermal evaporation onto a room-temperature substrate in a vacuum chamber with base pressure of 5.0 × 10 −9 Torr. Without breaking the vacuum, the Co (10 nm)/Au (7 nm) was then deposited by thermal evaporation at substrate temperature of 280 K to complete the formation of the top electrode in a crossbar configuration through the shadow mask. The thickness of layers were controlled by a quartz thickness monitor. The device area is ~200 μm × 50 μm. Device characterizations Atomic force microscopy topography images and PFM were taken using a Veeco Dimension 3100 at room temperature. The TEM samples were prepared by a FEI Dual-beam (Focus-Ion-Beam/SEM) system, and high-resolution TEM images were taken by a FEI Tecnai transmission electric microscope with beam energy of 200 kV. Radiant Premier II FE measuring system was used to detect the polarization-voltage loops of the devices at 50 Hz. Magnetometer measurements were carried out using a Quantum Design superconducting quantum interference device system. Magnetic fields were applied in the plane of the thin film. Transport measurements were carried out using a Quantum Design Physical Property Measurement System (PPMS) combined with a Keithley 2400 source meter at T =11 K. Magnetic fields were applied in the plane of the thin film. The MR is defined as: MR =( R antiparallel −R parallel )/R parallel , where R antiparallel is the junction resistance in the antiparallel magnetic configuration and R parallel is the resistance at the parallel configuration. The detailed MR measurement protocols are shown in Supplementary Fig. 2 and Supplementary Note 2 . How to cite this article: Sun, D. et al. Active control of magnetoresistance of organic spin valves using ferroelectricity. Nat. Commun. 5:4396 doi: 10.1038/ncomms5396 (2014).